Gene silencing by CRISPR interference in mycobacteria Recombination-based tools for introducing targeted genomic mutations in Mycobacterium tuberculosis are not efficient due to higher rate of illegitimate recombination compared with homologous DNA exchange. Moreover, involvement of multiple steps and specialized reagents make these tools cost ineffective. Here we introduce a novel clustered regularly interspaced short palindromic repeat (CRISPR) interference (CRISPRi) approach that efficiently represses expression of target genes in mycobacteria. CRISPRi system involves co-expression of the catalytically dead form of RNA-guided DNA endonuclease from the type II CRISPR system known as dCas9 and the small guide RNA specific to a target sequence, resulting in the DNA recognition complex that interferes with the transcription of corresponding DNA sequence. We show that co-expression of the codon-optimized dCas9 of S. pyogenes with sequence-specific guide RNA results in complete repression of individual or multiple targets in mycobacteria. CRISPRi thus offers a simple, rapid and cost-effective tool for selective control of gene expression in mycobacteria. M ycobacterium tuberculosis (Mtb), the causal agent of disease tuberculosis (TB) has latently infected ~2 billion people worldwide [1] . Despite clinical success in curing TB, it remains a major killer. A recent report by World Health Organization reveals that nearly 1.3 million people succumbed to TB and at least 8.6 million developed the disease in 2012 (ref. 1 ). Therefore, effective vaccines and drugs for reducing the global burden of TB are immediately required. Progress in identifying and characterizing appropriate vaccine candidates and drug targets has been severely impeded by a general lack of efficient tools for the directed inactivation of genes in Mtb. The most common approach for functional analysis of genes is to introduce genomic deletions by homologous recombination. Unfortunately, the existing techniques relying on recombination such as those employing non-replicating vectors [2] , long linear DNA fragments [3] , incompatible plasmids [4] , counterselectable marker SacB6 (ref. 5 ), specialized transducing mycobacteriophage carrying the allelic exchange substrate [6] and overexpression of mycobacteriophage-encoded recombination proteins [7] are not efficient in creating specific chromosomal mutations in mycobacterial genome. Importantly, none of these methods are suitable for targeting essential genes. With the advent of inducible promoters, the conditional gene expression technology was developed for functional characterization of mycobacterial genes that regulate essential cellular functions [8] , [9] . The inducible promoter can be implemented either to conditionally complement chromosomal gene disruption [10] or to replace the native promoter of a gene on the chromosome by a single crossover [11] . However, a major drawback of the promoter-swapping technique is its inability to provide the native expression level of a target gene in conditional mutant strain under permissive conditions. Recently, various other strategies were reported for targeted gene regulation in other microbial systems such as RNA interference, expression of engineered transcription activator-like effector proteins and interference by clustered regularly interspaced short palindromic repeat (CRISPR) sequences that need to be tested in mycobacterial species [12] , [13] , [14] . While RNA interference is restricted to particular organisms, custom DNA-binding proteins are difficult to implement because of high cost associated with their designing and testing [15] . Contrary to these, CRISPR interference (CRISPRi) approach offers a simple and cost-effective tool principally applicable to all microorganisms for targeted gene regulation [16] . CRISPR/Cas (CRISPR-associated proteins) system exists in majority of bacteria and archaea where it provides resistance to these organisms against the foreign DNA elements by selective cleavage [17] . CRISPR/Cas-mediated immunity to the foreign nucleic acids is a three-step process that begins with the adaptation stage at which small DNA fragments are integrated into the host genome between short DNA repeats with the help of the highly conserved Cas proteins, Cas1 and Cas2. As a result, an array of repeat sequences is created in the host chromosome interspersed by short, unique spacers. Selection of spacer precursors (proto-spacers) from the invading nucleic acids is achieved by unique proto-spacer adjacent motifs (PAMs) [18] . The second stage involves expression of the long primary transcript of a CRISPR locus known as pre-crRNA, which is processed into short crRNAs, either by a single endonuclease (such as Cas6 in Pyrococcus furiosus ) or by multi-protein complex (such as CRISPR-associated complex for antiviral defence (cascade) in Escherichia coli ) [19] , [20] , [21] . Subsequently, in the third and final stage, the mature crRNAs guide the respective complexes of Cas proteins to the complementary target sequences (either RNA or DNA) that match the spacers, adjacent to the respective PAM sequences, which leads to their cleavage. On the basis of arrangement of the cas genes, CRISPR/Cas system is classified into three different types [17] . Out of three different CRISPR systems, the type II CRISPR of Streptococcus pyogenes is the simplest one, which involves an endonuclease Cas9 and two RNAs, a mature crRNA and a partially complementary trans-acting RNA, for the RNA-guided repression of foreign DNAs [22] , [23] . Recently, it was shown that the requirement of two RNAs can be circumvented by the single custom-designed small guide RNA (sgRNA), which harbours required motifs for holding Cas9 endonuclease and simultaneous hybridization with the target DNA sequence [23] . As a consequence of the sgRNA–DNA base pairing, double-strand breaks in the target sequence are introduced by the associated Cas9 endonuclease ( Fig. 1a ). Other than sequence complementarity, the short PAM sequence 5′-NGG-3′ that is present next to the site of hybridization also plays an important role in determining specificity of CRISPR system [24] . Recently, a modified CRISPR system was developed for targeted gene regulation in E. coli by using the endonuclease-deficient Cas9, designated as dCas9 that contains two mutations—D10A and H840A—in the nuclease domains. The modified CRISPR system was termed as CRISPRi due to ability of the dCas9 to interfere with DNA transcription ( Fig. 1b ), which may repress gene expression by as many as thousand-fold [25] . 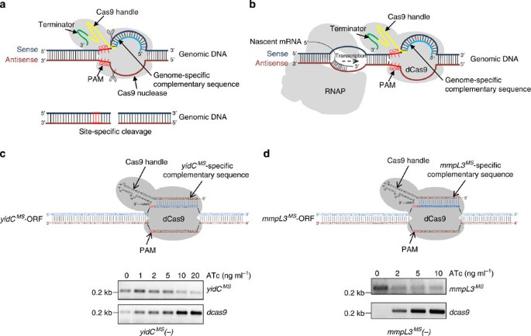Figure 1: Schematic of the CRISPRi approach. (a) Cartoon representation of CRISPR-mediated regulation of gene expression. The modified CRISPR system consists of two components: a ~150-kDa endonuclease, Cas9, and a designed sgRNA chimeric sequence. The sgRNAs comprises of three regions, a 20 nt complementary sequence (cyan), followed by 42 nt Cas9 handle (yellow) and a 40 nt transcription terminator (green), derived fromS. pyogenes. The wild-type Cas9 protein binds to the sgRNA and forms a protein–RNA complex. Regulation of gene expression by CRISPR is achieved when Cas9–sgRNA complex binds to specific DNA target adjacent to the proto-spacer adjacent motif (PAM, sequences are shown in red) by Watson–Crick base pairing between the sgRNA and the target DNA sequence, which results in cleavage of the DNA target due to the nuclease activity of the Cas9 protein. (b) Cartoon depicting regulation of gene expression by CRISPRi due to interference of RNAP transcription by nuclease-deficient dCas9. The nuclease-deficient dCas9 containing two substitutions in the nuclease domains (D10A and H840A) makes complex with sgRNA, which is targeted to specific DNA sequence. If the target DNA sequence belongs to the protein-coding region, the dCas9–sgRNA–DNA complex blocks the movement of RNAP and subsequent transcription elongation. (c,d) Silencing of genes by CRISPRi in Msm. Cartoon exhibiting binding ofyidCMS- (c) andmmpL3MS(d)-specific sgRNA–dCas9 complexes with the sense strand of the respective ORFs inyidCMS(−)andmmpL3MS(−)knockdown strains, respectively. Messenger RNAs extracted from these strains after 24 h of treatment with different ATc concentrations were subjected to complementary DNA (cDNA) synthesis. Equal amounts of cDNAs were subsequently used for PCR amplification of ~200-bp region of the respective ORFs by using specific forward and reverse primers (Supplementary Table 2). Expression was determined by visualizing intensities of amplicons on agarose gel that clearly indicates a dose-dependent repression of both the transcripts by dCas9 in the corresponding Msm strains. Data represent two experiments inc,d. Figure 1: Schematic of the CRISPRi approach. ( a ) Cartoon representation of CRISPR-mediated regulation of gene expression. The modified CRISPR system consists of two components: a ~150-kDa endonuclease, Cas9, and a designed sgRNA chimeric sequence. The sgRNAs comprises of three regions, a 20 nt complementary sequence (cyan), followed by 42 nt Cas9 handle (yellow) and a 40 nt transcription terminator (green), derived from S. pyogenes . The wild-type Cas9 protein binds to the sgRNA and forms a protein–RNA complex. Regulation of gene expression by CRISPR is achieved when Cas9–sgRNA complex binds to specific DNA target adjacent to the proto-spacer adjacent motif (PAM, sequences are shown in red) by Watson–Crick base pairing between the sgRNA and the target DNA sequence, which results in cleavage of the DNA target due to the nuclease activity of the Cas9 protein. ( b ) Cartoon depicting regulation of gene expression by CRISPRi due to interference of RNAP transcription by nuclease-deficient dCas9. The nuclease-deficient dCas9 containing two substitutions in the nuclease domains (D10A and H840A) makes complex with sgRNA, which is targeted to specific DNA sequence. If the target DNA sequence belongs to the protein-coding region, the dCas9–sgRNA–DNA complex blocks the movement of RNAP and subsequent transcription elongation. ( c , d ) Silencing of genes by CRISPRi in Msm. Cartoon exhibiting binding of yidC MS - ( c ) and mmpL3 MS ( d )-specific sgRNA–dCas9 complexes with the sense strand of the respective ORFs in yidC MS (−) and mmpL3 MS (−) knockdown strains, respectively. Messenger RNAs extracted from these strains after 24 h of treatment with different ATc concentrations were subjected to complementary DNA (cDNA) synthesis. 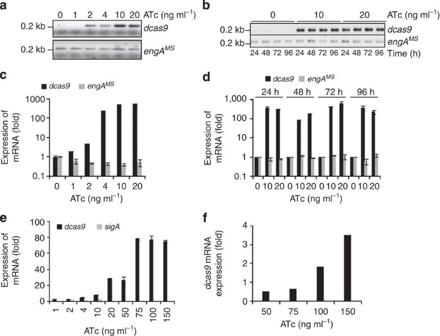Figure 2: Expression analysis ofdcas9in mycobacteria. (a–d) Analysis of ATc-inducibledcas9expression in Msm. Complementary DNAs were synthesized from Msm–dCas9 after treatment with different ATc concentrations and equal amounts of cDNAs were used for PCR amplification of ~200-bp region ofdcas9using gene-specific forward and reverse primers (Supplementary Table 2). Expression was determined by visualizing intensities of amplicons on agarose gel (a,b) or by quantitative real-time PCR (RT–PCR) (c,d). A dose-dependent induction ofdcas9expression was observed after ATc treatment (a,c), which was consistent over a period of 4 days (b,d), whereas expression of an unrelated gene,engAMSremained unaltered in these samples. (e) Analysis ofdcas9expression in BCG. Expression ofdcas9was analysed in BCG–dCas9 by RT–PCR after 2 days of treatment with different ATc concentrations. The graph shows a specific effect of ATc on the expression ofdcas9, while an unrelated control genesigAremains constant in all samples. (f) Stability ofdcas9expression in BCG. A modest change indcas9levels in BCG–dCas9 after 12 days of incubation with ATc in comparison with its expression after 2 days of ATc treatment indicates a stable expression ofdcas9. Data represent two experiments inaandb; mean±s.d. of multiple experiments is shown (n=3 inc,dande, andn=2 inf). Equal amounts of cDNAs were subsequently used for PCR amplification of ~200-bp region of the respective ORFs by using specific forward and reverse primers ( Supplementary Table 2 ). Expression was determined by visualizing intensities of amplicons on agarose gel that clearly indicates a dose-dependent repression of both the transcripts by dCas9 in the corresponding Msm strains. Data represent two experiments in c , d . Full size image Here we implement CRISPRi system in both the fast-growing M. smegmatis (Msm) and the slow-growing Mtb complex bacteria. A surveillance of mycobacterial genome reveals existence of the single CRISPR/Cas locus comprising of 9 genes, Rv2816c – Rv2824c that encode proteins of type III A system showing homology with Cas2, Cas1, Csm6, Csm5, Csm4, Csm3, Csm2, Cas10 and Cas6 proteins, respectively [26] . As the type II CRISPR/Cas system is absent in mycobacteria, we utilize codon-optimized dCas9 of S. pyogenes , which is stable for up to 2 weeks without any toxic or off-target effects in mycobacteria. Further, we construct an E. coli –mycobacteria shuttle plasmid to achieve expression of gene-specific complementary sequences next to the dCas9-binding region under the control of a tetracycline-inducible promoter, P myc1 tetO [27] . By using this approach, we are able to efficiently repress diverse sets of genes exhibiting a wide range of native expression levels in both the Msm and the Mtb complex bacteria. We also demonstrate that CRISPRi approach can simultaneously knockdown multiple genes in mycobacteria. Finally, by using CRISPRi system, we are able to rapidly test the gene essentiality in mycobacteria. Expression of codon-optimized dCas9 in mycobacteria To evaluate CRISPRi system in mycobacteria, we first examined expression of dCas9 in mycobacteria. For optimized expression in mycobacteria, a total of 191 codons of the original dcas9 of S. pyogenes were modified in such a way that corresponding amino acids remain unaltered ( Supplementary Fig. 1a,b ). Subsequently, the 4,107 base pair (bp) long codon-optimized dcas9 open reading frame (ORF) sequence flanked by Nde1–HindIII sites was commercially synthesized (Genscript) and cloned into an integrative plasmid pTetInt at the same sites under control of the P myc1 tetO promoter ( Supplementary Fig. 2a ). The resulting construct pTetInt– dcas9 was used to transform the fast-growing Msm mc 2 155, the slow-growing avirulent vaccine strain M. bovis BCG Pasteur (BCG) and the virulent Mtb strain H 37 Rv, respectively. The respective transformants were selected on 7H11 agar plates containing kanamycin after 7 (Msm–dCas9) or 21 days (BCG–dCas9 and Mtb–dCas9). Induction of dcas9 expression by a non-toxic tetracycline derivative, the anhydrotetracycline (ATc) was subsequently analysed in both the fast- and the slow-growing mycobacteria by real-time PCR (RT–PCR). Msm–dCas9 cultures treated for 24 h with different doses of ATc demonstrated the induction of dcas9 expression in a dose-dependent manner. However, dcas9 is not induced beyond 500-fold with ATc above 10 ng ml −1 ( Fig. 2a,c ). Next, we analysed the stability of dcas9 expression in Msm–dCas9 over a period of 4 days of growth in the presence of 10 or 20 ng ml −1 ATc. As shown in Fig. 2b,d , the levels of dcas9 is maintained in Msm at all time points. As dCas9 is a foreign protein, we also analysed the effect of dCas9 overexpression on bacterial growth. Growth of ATc-untreated or -treated Msm–dCas9 was monitored by measuring culture density at 600 nm (OD600). Our results demonstrated that ATc treatment up to 50 ng ml −1 does not affect in vitro growth of Msm–dCas9 ( Supplementary Fig. 3a ). Figure 2: Expression analysis of dcas9 in mycobacteria. ( a – d ) Analysis of ATc-inducible dcas9 expression in Msm. Complementary DNAs were synthesized from Msm–dCas9 after treatment with different ATc concentrations and equal amounts of cDNAs were used for PCR amplification of ~200-bp region of dcas9 using gene-specific forward and reverse primers ( Supplementary Table 2 ). Expression was determined by visualizing intensities of amplicons on agarose gel ( a , b ) or by quantitative real-time PCR (RT–PCR) ( c , d ). A dose-dependent induction of dcas9 expression was observed after ATc treatment ( a , c ), which was consistent over a period of 4 days ( b , d ), whereas expression of an unrelated gene, engA MS remained unaltered in these samples. ( e ) Analysis of dcas9 expression in BCG. Expression of dcas9 was analysed in BCG–dCas9 by RT–PCR after 2 days of treatment with different ATc concentrations. The graph shows a specific effect of ATc on the expression of dcas9 , while an unrelated control gene sigA remains constant in all samples. ( f ) Stability of dcas9 expression in BCG. A modest change in dcas9 levels in BCG–dCas9 after 12 days of incubation with ATc in comparison with its expression after 2 days of ATc treatment indicates a stable expression of dcas9 . Data represent two experiments in a and b ; mean±s.d. of multiple experiments is shown ( n =3 in c , d and e , and n =2 in f ). Full size image Next, the expression of dcas9 was assessed in BCG. It was observed that similar to Msm, BCG also exhibits a dose-dependent expression of dcas9 , although a minimum of 75 ng ml −1 ATc is required to obtain its peak expression in BCG ( Fig. 2e ). The quantitative RT–PCR estimation revealed that treatment of BCG–dCas9 with 75 ng ml −1 ATc for 2 days results in ~80-fold upregulation of dcas9 expression in comparison with its levels in the untreated culture ( Fig. 2e ). Further increasing the amount of inducer, however, does not enhance dcas9 expression. Moreover, expression of dcas9 is consistent in BCG for up to 2 weeks ( Fig. 2f ) and sustained dCas9 expression does not affect bacterial growth ( Supplementary Fig. 3b ) or gene expression profile, as observed by microarray ( Supplementary Table 1 and Supplementary Data 1 ). Overall, these observations demonstrate that dCas9 can be expressed consistently in mycobacteria without imposing any adverse effect on their in vitro growth. Construction of plasmid to express sgRNA in mycobacteria To test the utility of CRISPRi system in targeted gene regulation in mycobacteria, we constructed a replicative plasmid for the co-expression of gene-specific sgRNA with dCas9 in mycobacteria. For this, two complementary oligonucleotides namely gRNA_UP and gRNA_DN ( Supplementary Table 2 ) were synthesized and annealed together, which yielded a 100 bp-long DNA segment corresponding to the sgRNA cassette ( Supplementary Fig. 2b ). The resulting sgRNA cassette contains sites for cloning the target-specific complementary sequences followed by Cas9-binding hairpin sequence (Cas9 handle) and a transcriptional terminator derived from S. pyogenes (terminator) [23] , [25] ( Supplementary Fig. 2b ). The sgRNA cassette with SphI and HindIII overhangs at 5′ and 3′ ends, respectively, was then cloned at the same sites into a replicative plasmid pTetR downstream to P myc1 tetO promoter. The resulting plasmid was designated as pGrna ( Supplementary Fig. 2b–d ). For silencing the gene expression, target-specific short complementary oligonucleotide sequences ( Supplementary Table 2 ) were synthesized, annealed and cloned at unique SphI and AclI sites into pGrna as described in Methods. Consequently, on ATc treatment, mycobacterial cells harbouring pGrna derivatives express chimeric sgRNA molecules, each of which consists of three segments: a 20 nucleotide (nt) target-specific complementary region, a 42 nt Cas9 handle and a 40 nt transcription terminator. Effect of CRISPRi on repression of different Msm transcripts Next, we tested efficacy of CRISPRi approach in knocking-down the expression of genes in Msm. As depicted by the cartoon in Fig. 1b , we propose that CRISPRi blocks the transcription initiation or elongation by RNA polymerase (RNAP). Transcriptional repression by ATc was examined in mycobacteria harbouring pTetInt– dcas9 and pGrna derivatives. 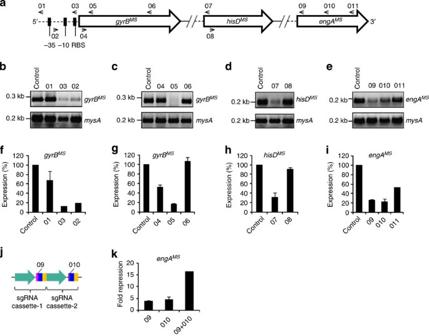Figure 3: Determinants of CRISPRi efficiency in mycobacteria. (a) Arrangement of mycobacterial genes and positions of different sgRNAs. Mycobacterial genes at different loci are represented by hollow arrows pointed in the direction of 5′→3′ and separated by parallel lines. The broken horizontal lines correspond to the respective 5′-UTRs. The vertical bars in the 5′-UTR ofgyrBMSrepresent ribosome-binding site (RBS), −10 and −35 boxes of its promoter, respectively. Positions of different sgRNA oligonucleotides (O1–O11) are marked by small arrows pointed in the direction of 5′→3′. (b–i) Influence of sgRNA positions and directions on the silencing efficiency of CRISPRi in mycobacteria. Expression of dCas9 in Msm either alone (control) or together with the respective sgRNAs (O1–O11) was achieved by 24 h of treatment with 10 ng ml−1ATc, and its effect on the expression levels of the corresponding transcripts was determined. Equal amounts of cDNAs prepared from the control and the respective knockdown strains of Msm were used for PCR amplification of ~200-bp region of respective ORFs by using specific forward and reverse primers (Supplementary Table 2). Expression of a transcript in the corresponding knockdown strain relative to its expression in the control was determined by visualizing intensities of the respective amplicons on 1% agarose gel (b–e) and by quantitative RT–PCR using normalization tomysAtranscript levels (f–i). (j,k) Influence of multiple sgRNAs on silencing efficiency of CRISPRi. (j) Cartoon representing the arrangement of twoengAMS-specific sgRNA cassettes in pGrna plasmid. Each sgRNA cassette comprises of an ATc-inducible promoter,Pmyc1tetO(green arrows) followed by target-specific sgRNA oligonucleotides O9 (pink) or O10 (magenta), Cas9 handle (blue) and a transcription terminator (orange) derived fromS. pyogenes. (k) Analysis ofengAMStranscript levels in Msm expressing dCas9 either alone (control) or together with the O9–O10 sgRNAs by quantitative RT–PCRs. Fold repression inkrepresents the downregulation ofengAMStranscript levels in the respective knockdown strains relative to its expression in control; the values were obtained using normalization tomysAtranscript levels, which remained constant in the two strains. Data represent two experiments inb–e; mean ±s.d. of three measurements is shown inf–iandk. Various genes exhibiting a range of expression levels in wild-type bacteria ( Supplementary Table 3 ) were targeted to evaluate the efficacy of CRISPRi approach in silencing their respective expression levels in Msm. The optimum concentration of ATc for the maximum repression was determined using one of the highly expressed transcripts MSMEG_6942 ( yidC MS ) and a moderately expressed transcript MSMEG_0250 ( mmpL3 MS ), respectively ( Supplementary Table 3 ). As sgRNAs targeting the sense strand of coding sequences exhibit better silencing efficiency than those binding to the antisense strand [25] , we began our analysis with the co-expression of dCas9 and a 20-bp sgRNA sequence complementary to the sense strand of either the yidC MS - or mmpL3 MS -coding sequences. Expression levels of these genes in the respective knockdown strains yidC MS (−) and mmpL3 MS (−) were examined after 24 h of treatment with different ATc concentrations ( Fig. 1c,d ). It was observed that yidC MS expression is gradually downregulated with increasing ATc amounts ( Fig. 1c ). By quantitative RT–PCR it was estimated that expression of yidC MS is reduced by 0%, 52%, 65%, 85% and 94% in the yidC MS (−) treated with 1, 2, 4, 10 and 20 ng ml −1 ATc, respectively, in comparison with its levels in the untreated bacteria. In contrast, expression of dcas9 is gradually increased by up to 324-fold after treatment with 20 ng ml −1 ATc ( Fig. 1c ). Similar result was also obtained when a relatively less-abundant transcript of mmpL3 MS was targeted for CRISPRi-mediated repression. Our results demonstrated that the expression of mmpL3 MS is suppressed by >90% in mmpL3 MS (−) strain after incubating with 10 ng ml −1 ATc for 24 h ( Fig. 1d ). Determinants of CRISPRi efficiency in mycobacteria To establish CRISPRi as the general tool for effective repression of genes in mycobacteria, we sought to determine roles of sequence complementarity and position of sgRNA on silencing efficiency of CRISPRi. Three different genes, MSMEG_0005 ( gyrB MS ), MSMEG_3205 ( hisD MS ) and MSMEG_3738 (e ngA MS ), were targeted for such analyses ( Supplementary Table 3 ). The 20-bp sequences binding to the antisense strand (O2, O4 and O8) or to the sense strand (O1, O3, O5, O6, O7, O9, O10 and O11) at different positions in the 5′-untranslated region (5′-UTR; O1–O3) or in the coding region (O4–O11) of these genes were individually expressed as chimeric sgRNA in Msm overexpressing dCas9 under the control of P myc1 tetO promoter ( Supplementary Table 2 ). The effect of sgRNA–dCas9 co-expression on the respective transcript levels was subsequently analysed by RT–PCR ( Fig. 3a–i ). Our results demonstrated that sgRNAs targeting the coding region are effective (>80% repression) only if they bind to the sense strand ( Fig. 3 ; O5, O7, O9 and O10), whereas those targeting the antisense strand in the coding region do not silence the gene expression ( Fig. 3 ; O4 and O8). Interestingly, such distinction in the efficiency of sgRNA does not exist when the 5′-UTR is targeted ( Fig. 3 ; O2 and O3). We observed that sgRNAs binding to either the antisense (O2) or the sense (O3) strand of 5′-UTR are equally effective in silencing the expression ( Fig. 3a,b,f ). Another factor that determines the efficacy of CRISPRi is the distance from the transcription start site at which sgRNA binds, either in the 5'-UTR or in the coding region. As shown in Fig. 3 , sequences ~100 bp upstream of −35 box in the promoter region (O1), as well as those towards 3′ end of the coding sequences (O6 and O11) are ineffective in modulating expression of the respective transcripts. Figure 3: Determinants of CRISPRi efficiency in mycobacteria. ( a ) Arrangement of mycobacterial genes and positions of different sgRNAs. Mycobacterial genes at different loci are represented by hollow arrows pointed in the direction of 5′→3′ and separated by parallel lines. The broken horizontal lines correspond to the respective 5′-UTRs. The vertical bars in the 5′-UTR of gyrB MS represent ribosome-binding site (RBS), −10 and −35 boxes of its promoter, respectively. Positions of different sgRNA oligonucleotides (O1–O11) are marked by small arrows pointed in the direction of 5′→3′. ( b – i ) Influence of sgRNA positions and directions on the silencing efficiency of CRISPRi in mycobacteria. Expression of dCas9 in Msm either alone (control) or together with the respective sgRNAs (O1–O11) was achieved by 24 h of treatment with 10 ng ml −1 ATc, and its effect on the expression levels of the corresponding transcripts was determined. Equal amounts of cDNAs prepared from the control and the respective knockdown strains of Msm were used for PCR amplification of ~200-bp region of respective ORFs by using specific forward and reverse primers ( Supplementary Table 2 ). Expression of a transcript in the corresponding knockdown strain relative to its expression in the control was determined by visualizing intensities of the respective amplicons on 1% agarose gel ( b – e ) and by quantitative RT–PCR using normalization to mysA transcript levels ( f – i ). ( j , k ) Influence of multiple sgRNAs on silencing efficiency of CRISPRi. ( j ) Cartoon representing the arrangement of two engA MS -specific sgRNA cassettes in pGrna plasmid. Each sgRNA cassette comprises of an ATc-inducible promoter, P myc1 tetO (green arrows) followed by target-specific sgRNA oligonucleotides O9 (pink) or O10 (magenta), Cas9 handle (blue) and a transcription terminator (orange) derived from S. pyogenes . ( k ) Analysis of engA MS transcript levels in Msm expressing dCas9 either alone (control) or together with the O9–O10 sgRNAs by quantitative RT–PCRs. Fold repression in k represents the downregulation of engA MS transcript levels in the respective knockdown strains relative to its expression in control; the values were obtained using normalization to mysA transcript levels, which remained constant in the two strains. Data represent two experiments in b – e ; mean ±s.d. of three measurements is shown in f – i and k . Full size image Further, we investigated whether simultaneous expression of multiple sgRNAs targeting the same transcript results in better silencing. Two sgRNAs, O9 and O10, recognizing different positions of the engA MS -coding sequence were co-expressed in Msm–dCas9 and their effect on engA MS transcript levels was examined by RT–PCR ( Fig. 3a,j,k ). Our observations that O9 and O10, each causing ~4-fold repression of engA MS , together suppress its expression by 16-fold, clearly suggest a cumulative effect of multiple sgRNAs on silencing efficiency of CRISPRi ( Fig. 3k ). Suppression of protein expression in Msm by CRISPRi To test whether the CRISPRi approach is equally efficient at the protein level, we determined the levels of YidC MS and EngA MS proteins in yidC MS (−) and in Msm–dCas9 overexpressing the O9 sgRNA (designated as engA MS (−) ), respectively ( Figs 1c and 3a ). Expression of these proteins was observed by immunoblotting using the whole-cell extract prepared from the respective strains after 24 h of treatment with various ATc concentrations ( Fig. 4 ). 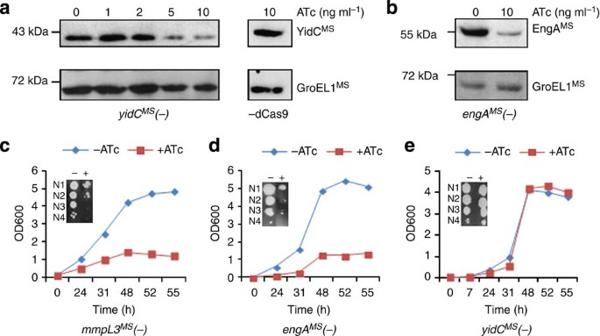Figure 4: Silencing of protein expression by CRISPRi in Msm. (a,b) Effect of CRISPRi on protein synthesis in Msm. Whole-cell extracts of the respective Msm strains were prepared after 24 h of treatment either with different (a) or with fixed ATc concentrations (b), and subjected to immunoblot analyses using specific antibodies, which show that expression of the respective proteins and not of an unrelated protein GroEL1 disappears following ATc treatment in a dose-dependent manner. (c–e) Influence of CRISPRi-mediated silencing of genes onin vitrogrowth of Msm.In vitrogrowth was determined by measuring OD600 of individual knockdown strains, in the presence (+) or the absence (−) of 50 ng ml−1ATc. Also, an aliquot of each culture, after 24 h of growth, was subjected to 10-fold serial dilution and spotted on 7H11 agar plates with (+) or without (−) 10 ng ml−1ATc; dilutions are as follows: N1: 10−1, N2: 10−2, N3: 10−3and N4: 10−4, respectively (see insets). These results clearly show that likemmpL3MS,engAMSis essential in Msm. Interestingly, another geneyidCMS, predicted to be essential, was found dispensable forin vitrogrowth of fast-growing Msm. Data represent two experiments inaandb; mean±s.d. of three measurements is shown inc–e. Figure 4 demonstrates that CRISPRi efficiently downregulates the expression of YidC MS and EngA MS proteins in the respective knockdown strains ( Fig. 4a,b ). By densitometric analysis, it was estimated that expression of YidC MS and EngA MS is reduced by 75% and 90% in the yidC MS (−) and the engA MS (−) strains, respectively, after 24 h of treatment with 10 ng ml −1 ATc ( Fig. 4a,b ). Conversely, there was no effect of ATc treatment on the expression of YidC MS in Msm–pGrna– yidC MS lacking dCas9 (−dCas9), which indicates a direct effect of dCas9 on the expression of these proteins in Msm ( Fig. 4a ). Figure 4: Silencing of protein expression by CRISPRi in Msm. ( a , b ) Effect of CRISPRi on protein synthesis in Msm. Whole-cell extracts of the respective Msm strains were prepared after 24 h of treatment either with different ( a ) or with fixed ATc concentrations ( b ), and subjected to immunoblot analyses using specific antibodies, which show that expression of the respective proteins and not of an unrelated protein GroEL1 disappears following ATc treatment in a dose-dependent manner. ( c – e ) Influence of CRISPRi-mediated silencing of genes on in vitro growth of Msm. In vitro growth was determined by measuring OD600 of individual knockdown strains, in the presence (+) or the absence (−) of 50 ng ml −1 ATc. Also, an aliquot of each culture, after 24 h of growth, was subjected to 10-fold serial dilution and spotted on 7H11 agar plates with (+) or without (−) 10 ng ml −1 ATc; dilutions are as follows: N1: 10 −1 , N2: 10 −2 , N3: 10 −3 and N4: 10 −4 , respectively (see insets). These results clearly show that like mmpL3 MS , engA MS is essential in Msm. Interestingly, another gene yidC MS , predicted to be essential, was found dispensable for in vitro growth of fast-growing Msm. Data represent two experiments in a and b ; mean±s.d. of three measurements is shown in c – e . Full size image Gene silencing in Mtb complex bacteria by CRISPRi As Msm and Mtb complex bacteria differ in their metabolism, it is prudent to evaluate the efficacy of CRISPRi approach in slow-growing mycobacterial species as well. Seven genes that exhibit a range of expression levels in Mtb were selected to analyse the efficiency of CRISPRi in silencing their expression in slow-growing mycobacteria; these include Rv1713 ( engA ), Rv2150c ( ftsZ ), Rv2460c ( clpP2 ), Rv3417c ( groEL1 ), Rv3418c ( groES ), Rv3596c ( clpC1 ) and Rv3921c ( yidC ) ( Supplementary Table 3 ). On the basis of above results, we targeted the sense strand of coding regions near the transcription start site of these genes. A 20-bp complementary sequence specific to each of these targets ( Supplementary Table 2 ) was first cloned into pGrna, which was then transformed into the Mtb–dCas9 and the BCG–dCas9 strains, respectively. The dCas9-overexpressing mycobacteria harbouring empty pGrna plasmid were simultaneously used as controls. To establish the conditions for maximum suppression, expression of yidC messenger RNA (mRNA) was first analysed in BCG–dCas9 harbouring either pGrna (control) or pGrna- yidC ( yidC(−) ), after 2 days of growth in the absence or the presence of different ATc concentrations. The semiquantitative RT–PCR results demonstrate that yidC transcript levels are gradually diminished in the yidC(−) knockdown strain in an ATc dose-dependent manner ( Fig. 5a ). Quantitative estimation by densitometric analysis revealed that expression of yidC is reduced by >90% in yidC(−) , after treatment with 100 ng ml −1 ATc. Importantly, yidC expression does not change in the control strain lacking yidC -specific sgRNA, under similar conditions ( Fig. 5a ). Further, the level of an unrelated gene sigA remains constant in these samples, which indicates equal loading of samples on the agarose gel ( Fig. 5a ). Overall, these results suggest that CRISPRi technique is highly specific and relies on expression of the target-specific sgRNAs for effective silencing. 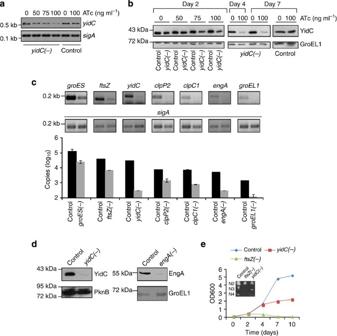Figure 5: Silencing of genes by CRISPRi in Mtb complex bacteria. (a,b) Effect of CRISPRi on expression of genes in BCG. Expression ofyidCtranscript (a) or YidC protein (b) was analysed in theyidC(−)strain of BCG after 2 days of treatment with different ATc concentrations. Note thatyidCtranscript levels are decreased with increasing ATc concentrations inyidC(−)but not in control strain containing empty pGrna plasmid. Effect of CRISPRi on suppression of YidC protein was more prominent after 4 or 7 days of treatment with 100 ng ml−1ATc (b). (c,d) Effect of CRISPRi on repression of the differentially abundant transcripts in Mtb. Seven genes encompassing a range of expression levels in Mtb were selected to evaluate the efficacy of CRISPRi in silencing the expression of differentially abundant transcripts present at various loci in Mtb. Expression of various genes was analysed at the RNA (c) and at the protein (d) level in the control and the respective knockdown strains after treatment with 100 ng ml−1ATc for 4 days. Number of copies of each transcript per 50 ng RNA was estimated by performing the quantitative PCR using serial dilutions of genomic DNA template and gene-specific forward and reverse primers that amplify ~200-bp sequence (Supplementary Table 2). As can be seen, under these experimental conditions, a significant repression of target genes (>80%) was achieved irrespective of their abundance (c–d). Expressions ofsigA(a,c), GroEL1 (b,d) and PknB (d) are shown to demonstrate equal loading. (e) Effect of CRISPRi-mediated silencing of essential genes onin vitrogrowth of Mtb.In vitrogrowth was determined by measuring OD600 of the control and the individual knockdown strains, treated with 100 ng ml−1ATc. Also, an aliquot of each of these cultures, after 48 h of treatment with 100 ng ml−1ATc, was subjected to 10-fold serial dilution and spotted on 7H11-OADC agar plates to monitor growth after 4 weeks; dilutions are as follows: N2: 10−2, N3: 10−3and N4: 10−4, respectively (see insets). These results demonstrate that in contrast to Msm,yidCis essential in Mtb. Data represent two experiments ina–d; mean±s.d. of three measurements is shown ine. Figure 5: Silencing of genes by CRISPRi in Mtb complex bacteria. ( a , b ) Effect of CRISPRi on expression of genes in BCG. Expression of yidC transcript ( a ) or YidC protein ( b ) was analysed in the yidC(−) strain of BCG after 2 days of treatment with different ATc concentrations. Note that yidC transcript levels are decreased with increasing ATc concentrations in yidC(−) but not in control strain containing empty pGrna plasmid. Effect of CRISPRi on suppression of YidC protein was more prominent after 4 or 7 days of treatment with 100 ng ml −1 ATc ( b ). ( c , d ) Effect of CRISPRi on repression of the differentially abundant transcripts in Mtb. Seven genes encompassing a range of expression levels in Mtb were selected to evaluate the efficacy of CRISPRi in silencing the expression of differentially abundant transcripts present at various loci in Mtb. Expression of various genes was analysed at the RNA ( c ) and at the protein ( d ) level in the control and the respective knockdown strains after treatment with 100 ng ml −1 ATc for 4 days. Number of copies of each transcript per 50 ng RNA was estimated by performing the quantitative PCR using serial dilutions of genomic DNA template and gene-specific forward and reverse primers that amplify ~200-bp sequence ( Supplementary Table 2 ). As can be seen, under these experimental conditions, a significant repression of target genes (>80%) was achieved irrespective of their abundance ( c – d ). Expressions of sigA ( a , c ), GroEL1 ( b , d ) and PknB ( d ) are shown to demonstrate equal loading. ( e ) Effect of CRISPRi-mediated silencing of essential genes on in vitro growth of Mtb. In vitro growth was determined by measuring OD600 of the control and the individual knockdown strains, treated with 100 ng ml −1 ATc. Also, an aliquot of each of these cultures, after 48 h of treatment with 100 ng ml −1 ATc, was subjected to 10-fold serial dilution and spotted on 7H11-OADC agar plates to monitor growth after 4 weeks; dilutions are as follows: N2: 10 −2 , N3: 10 −3 and N4: 10 −4 , respectively (see insets). These results demonstrate that in contrast to Msm, yidC is essential in Mtb. Data represent two experiments in a – d ; mean±s.d. of three measurements is shown in e . Full size image Next, we analysed expression of YidC protein by immunoblotting of whole-cell extracts prepared from control and yidC(−) strains of BCG after 2, 4 and 7 days of treatment with various ATc concentrations. We observed that expression of YidC in yidC(−) is reduced in an ATc dose-dependent manner following 2 days of treatment and a maximum effect is obtained with 100 ng ml −1 ATc, which leads to ~50% reduction in expression ( Fig. 5b ). Remarkably, YidC expression is reduced by 85% and 92% in yidC(−) after subsequent incubations for 4 or 7 days, respectively, with 100 ng ml −1 ATc ( Fig. 5b ). In contrast, expression of YidC does not alter under these conditions in the control BCG strain, which corroborates the role of sgRNA sequences in determining the specificity of dCas9-mediated suppression of gene expression in mycobacteria ( Fig. 5b ). On the basis of these observations, we next analysed the effect of CRISPRi on expression of rest of the genes in virulent Mtb H 37 Rv after 4 days of treatment with 100 ng ml −1 ATc ( Fig. 5c,d ). It was observed that ATc treatment results in significant loss of expression of engA (94%), ftsZ (82%), clpP2 (81%), groEL1 (91%), groES (80%), clpC1 (89%) and yidC (99%) transcripts in the Mtb H 37 Rv-dCas9 harbouring pGrna- engA ( engA(−) ), pGrna- ftsZ ( ftsZ(−) ), pGrna- clpP2 ( clpP2(−) ), pGrna- groEL1 ( groEL1(−) ), pGrna- groES ( groES(−) ), pGrna- clpC1 ( clpC1(−) ) and pGrna- yidC ( yidC(−) ), respectively, in comparison with their expression in the control Mtb–dCas9 strain ( Fig. 5c ). Notably, the control Mtb H37Rv-dCas9 harbouring empty pGrna plasmid exhibits wild-type levels of expression of these transcripts under similar conditions. Moreover, expression of a housekeeping gene sigA remains constant in both the control and the knockdown strains ( Fig. 5c ). Similar to these results, we observed that CRISPRi is highly efficient in suppressing the expression of proteins. Expression of EngA and YidC in engA(−) and yidC(−) strains, respectively, was compared with their respective levels in the control Mtb, after 4 days of treatment with 100 ng ml −1 ATc. Figure 5d shows that both the proteins are completely suppressed in the respective knockdown strains, whereas unrelated proteins PknB or GroEL1 remain constant in both the control and knockdown strains ( Fig. 5d ). Overall, these results clearly demonstrate that CRISPRi approach is highly effective in knocking-down the expression of genes in mycobacteria both at the mRNA and at the protein levels. Assessment of gene essentiality in mycobacteria by CRISPRi One of the major strengths of CRISPRi approach is the ease with which genes can be repressed irrespective of their requirement for replication of mycobacteria in synthetic culture media. As a result, CRISPRi can be a valuable tool in identifying the essential genes in virulent Mtb that may be subsequently exploited as potential drug targets. To explore this attribute of CRISPRi, we determined the requirement of putative essential genes engA and yidC in both Msm and Mtb ( Figs 4c–e and 5e ). Concurrently, we also targeted known essential genes encoding cell wall component, MmpL3 and cell division protein FtsZ, respectively, which served as controls. In vitro growth was assessed by measuring OD600 of cultures at regular intervals, as well as by spotting serial dilutions of bacterial cultures on 7H11 agar plates supplemented with or without ATc, as described in Methods. Figure 4 demonstrates that repression of engA MS results in severely attenuated growth of Msm, which is similar to that of mmpL3 MS knockdown strain. Spotting of 10-fold serial dilutions of cultures on 7H11 plates revealed that growth of engA MS (−) strain is reduced by >1,000-fold in the presence of ATc, thus indicating the essential requirement of EngA in Msm as hypothesized earlier [28] ( Fig. 4c,d ). Conversely, repression of yidC does not affect growth of Msm in both 7H9 broth and on 7H11 agar media ( Fig. 4e ). Interestingly, when growth profiles of control, yidC(−) and ftsZ(−) strains of Mtb H 37 Rv were compared in the presence of ATc, it was observed that in contrast to Msm, YidC is required for in vitro growth of Mtb H 37 Rv both in 7H9 broth and on 7H11 agar media ( Fig. 5e ). Similar effect on growth was also observed after suppression of ftsZ in Mtb H 37 Rv, which exhibited >100-fold loss in colony-forming unit on 7H11 agar plates supplemented with 100 ng ml −1 ATc in comparison with control strain, which was unaffected by ATc treatment ( Fig. 5e and Supplementary Fig. 3b ). Evaluation of CRISPRi approach in silencing the operon To test the efficacy of CRISPRi in silencing the operon expression in mycobacteria, we explored the gyrB MS -gyrA MS and groES-groEL1 operons in which gyrA MS and groEL1 are positioned downstream to gyrB MS and groES , respectively [29] , [30] . Transcript levels of the gyrA MS were determined in the Msm–dCas9 strain co-expressing different sgRNAs O1–O5 that target different positions of gyrB MS locus ( Fig. 6a ). RT–PCR results demonstrated that similar to the gyrB MS , expression of the gyrA MS transcript is perturbed in the presence of O2, O3 and O5 sgRNAs. By quantitative RT–PCR, it was observed that in Msm–dCas9 expressing O2, O3 and O5 sgRNAs the gyrA MS expression is reduced to 25%, 12% and 14%, respectively, of its expression level in the control strain ( Fig. 6a ). In contrast, the O1 and O4 sgRNA sequences that were ineffective in modulating the expression of gyrB MS show no effect on the expression of gyrA MS transcript levels as well ( Fig. 6a ). Similar effect was observed with CRISPRi-targeting groES on the expression of downstream gene groEL1 in Mtb, which exhibits >90% reduction in groES(−) strain ( Fig. 6b ). 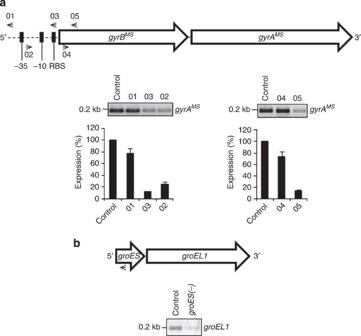Figure 6: Repression of operon expression by CRISPRi in mycobacteria. (a,b) Effect of CRISPRi on repression ofgyrAMSandgroEL1ingyrBMS-gyrAMS(a) andgroES-groEL1(b) operons, respectively. Arrangement of genes in different operons are represented by hollow arrows pointed in the direction of 5′→3′. The broken horizontal lines correspond to the respective 5′-UTRs. The vertical bars in the 5′-UTR ofgyrBMSrepresent ribosome-binding site (RBS), −10 and −35 boxes of its promoter, respectively. Positions of different sgRNA oligonucleotides are marked by small arrows pointed in the direction of 5′→3′. Expression of dCas9 either alone (control) or together with the respective sgRNAs was achieved in Msm by 24 h of treatment with 10 ng ml−1ATc (a) and in Mtb by 96 h of treatment with 100 ng ml−1ATc (b), respectively. Silencing of transcripts in the corresponding knockdown strains was determined by both the semiquantitative and the quantitative RT–PCRs, as described above. These results demonstrate that sgRNAs targeting the upstream genes of operon simultaneously repress the expression of downstream genes. Data represent two experiments inaandb; mean±s.d. of two measurements is shown in a. Figure 6: Repression of operon expression by CRISPRi in mycobacteria. ( a , b ) Effect of CRISPRi on repression of gyrA MS and groEL1 in gyrB MS -gyrA MS ( a ) and groES-groEL1 ( b ) operons, respectively. Arrangement of genes in different operons are represented by hollow arrows pointed in the direction of 5′→3′. The broken horizontal lines correspond to the respective 5′-UTRs. The vertical bars in the 5′-UTR of gyrB MS represent ribosome-binding site (RBS), −10 and −35 boxes of its promoter, respectively. Positions of different sgRNA oligonucleotides are marked by small arrows pointed in the direction of 5′→3′. Expression of dCas9 either alone (control) or together with the respective sgRNAs was achieved in Msm by 24 h of treatment with 10 ng ml −1 ATc ( a ) and in Mtb by 96 h of treatment with 100 ng ml −1 ATc ( b ), respectively. Silencing of transcripts in the corresponding knockdown strains was determined by both the semiquantitative and the quantitative RT–PCRs, as described above. These results demonstrate that sgRNAs targeting the upstream genes of operon simultaneously repress the expression of downstream genes. Data represent two experiments in a and b ; mean±s.d. of two measurements is shown in a. Full size image Suppression of multiple targets in mycobacteria by CRISPRi As CRISPRi blocks mRNA transcript synthesis by stalling the RNAP in a sequence-specific manner, we examined if more than one target sequence can be simultaneously repressed. To achieve this goal, sgRNAs complementary to gyrA MS -coding ( Supplementary Table 2 ) and engA MS (O9)-coding sequences, respectively, were cloned under the regulation of P myc1 tetO promoter in pGrna plasmid ( Fig. 7a ), which was then transformed into Msm–dCas9 resulting into a strain gyrA MS (−) / engA MS (−). Expression of gyrA MS and engA MS was subsequently analysed in the double knockdown strain of Msm after 24 h of treatment with 10 ng ml −1 ATc by RT–PCR, as described above. As demonstrated in Fig. 7b , ATc treatment upregulates the expression of dcas9 , whereas there is no change in the level of the control gene mysA in gyrA MS (−) / engA MS (−) strain ( Fig. 7b ). In contrast, expression of both the gyrA MS , as well as the engA MS is remarkably reduced in the ATc-treated cultures to 30% and 11%, respectively, of their respective expression levels in the ATc-untreated cultures ( Fig. 7b,c ). These results thus clearly demonstrate that CRISPRi approach is instrumental in modulating the expression of multiple genes in mycobacteria. 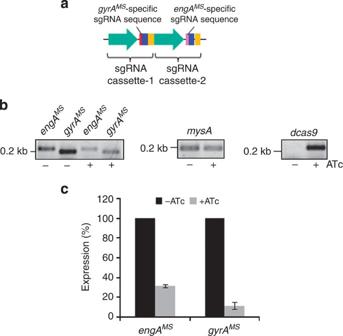Figure 7: Silencing of multiple genes by CRISPRi in mycobacteria. (a) Cartoon representing the arrangement of two sgRNA cassettes specific togyrAMSandengAMS, respectively, in pGrna plasmid. Each sgRNA cassette comprises ofPmyc1tetOpromoter (green arrows) followed bygyrAMS-specific (red) orengAMS-specific (pink) sgRNA oligonucleotides, Cas9 handle (blue) and a transcription terminator (orange) derived fromS. pyogenes. (b,c) Analysis ofgyrAMSandengAMStranscript levels in double knockdown strain,gyrAMS(−)/engAMS(−). Complementary DNAs were synthesized using mRNA ofgyrAMS(−)/engAMS(−)strain cultured in the absence (−) or the presence (+) of 10 ng ml−1ATc for 24 h. Equal amounts of cDNAs were subsequently used for PCR amplification of ~200-bp region of respective ORFs by using specific forward and reverse primers (Supplementary Table 2). Expression of transcripts in the ATc-treated cultures relative to their expression in untreated samples was determined by visualizing intensities of amplicons on agarose gel (b) or by quantitative real-time PCR (RT–PCR) (c) using normalization tomysAtranscript levels, which remains constant in the two strains. As shown, levels of bothgyrAMSandengAMSare significantly reduced subsequent to ATc treatment. Data represent two experiments in b; mean ±s.d. of three measurements is shown in c. Figure 7: Silencing of multiple genes by CRISPRi in mycobacteria. ( a ) Cartoon representing the arrangement of two sgRNA cassettes specific to gyrA MS and engA MS , respectively, in pGrna plasmid. Each sgRNA cassette comprises of P myc1 tetO promoter (green arrows) followed by gyrA MS -specific (red) or engA MS -specific (pink) sgRNA oligonucleotides, Cas9 handle (blue) and a transcription terminator (orange) derived from S. pyogenes . ( b , c ) Analysis of gyrA MS and engA MS transcript levels in double knockdown strain, gyrA MS (−) / engA MS (−) . Complementary DNAs were synthesized using mRNA of gyrA MS (−) / engA MS (−) strain cultured in the absence (−) or the presence (+) of 10 ng ml −1 ATc for 24 h. Equal amounts of cDNAs were subsequently used for PCR amplification of ~200-bp region of respective ORFs by using specific forward and reverse primers ( Supplementary Table 2 ). Expression of transcripts in the ATc-treated cultures relative to their expression in untreated samples was determined by visualizing intensities of amplicons on agarose gel ( b ) or by quantitative real-time PCR (RT–PCR) ( c ) using normalization to mysA transcript levels, which remains constant in the two strains. As shown, levels of both gyrA MS and engA MS are significantly reduced subsequent to ATc treatment. Data represent two experiments in b; mean ±s.d. of three measurements is shown in c. Full size image Despite the availability of the genome sequence since 1998, functions of a quarter of ~4,000 predicted ORFs of Mtb have remained uncharacterized [31] . Moreover, ~5% of the uncharacterized hypothetical proteins are predicted essential for mycobacterial growth in the synthetic culture media by transposon site hybridization analysis [32] , [33] . Hence, methods that can feasibly disrupt the expression of ORFs in Mtb will expedite the functional characterization of these hypothetical proteins, some of which may also be explored as potential drug targets. Here we have introduced a simple approach of gene silencing in mycobacteria by using a derivative of RNA-guided DNA endonuclease of type II CRISPR system known as dCas9 that lacks the nuclease activity. While existing techniques rely on laborious and costly genomic engineering procedures, gene knockdown with CRISPRi simply requires co-expression of dCas9 and short complementary oligonucleotide sequences, thus making this tool highly efficient. As Mtb lacks Cas9, we used dCas9 of S. pyogenes , a Gram-positive bacterium. We inclined to use ATc-inducible promoter to achieve controlled expression of target genes. Indeed, it was observed that dcas9 is expressed in an ATc dose-dependent manner in both the fast- and the slow-growing mycobacteria, albeit the requirement of inducer to achieve the maximum expression was different for both the species ( Fig. 2 ), which could be due to differential regulation of P myc1 tetO promoter by TetR in the two organisms [27] . However, despite this fact, dcas9 expression was consistent for >20 generations in Msm and for >10 generations in BCG, when supplemented with ATc at regular intervals ( Fig. 2b,d,f ). Further, overexpression of dCas9 does not lead to toxicity in both Msm and Mtb complex bacteria ( Supplementary Fig. 3 ). Notably, we sought to assess CRISPRi system particularly against essential genes that cannot be feasibly disrupted by conventional recombination-based tools. A total of 13 genes across a broad range of expression levels were targeted in evaluating the silencing efficiency of CRISPRi. The system was first optimized with Msm genes that exhibit relatively higher expression than their counterparts from slow-growing Mtb ( Supplementary Table 3 ). Different positions of sgRNA target sequences were carefully selected such that they are flanked by a PAM, 5′-NGG-3′, as CRISPRi is inefficient on sequences lacking PAM [25] . In addition, the minimum length of 20 bp of sgRNAs was used based on the previous report [25] . Our observation that sgRNA targeting either strand in the 5′-UTR exhibits comparable suppression (O2, O3, Fig. 3 ) suggests that dCas9 interferes with binding of the RNAP to the respective promoter sequence, which involves both the strands. This is also corroborated by the fact that sequences upstream to the core promoter region (O1) that are not recognized by RNAP [34] , exhibit no effect in mediating suppression by dCas9 binding ( Fig. 3 ). Conversely, the sgRNAs targeting the coding sequences work only if they bind to the sense strand (O5, O7, O9 and O10, Fig. 3 ), whereas those binding the antisense strand are inefficient in silencing expression of the respective transcripts (O4 and O8). Although the underlying cause for such distinction is not known, we anticipate this could be due to dislocation of sgRNA–dCas9 complexes facing towards the direction of RNAP movement because of its helicase activity. Interestingly, the strength of inhibition is increased by increasing the number of sgRNA targets on a transcript ( Fig. 3j,k ). Figures 1 and 3 illustrate that CRISPRi suppresses synthesis of mRNA transcripts irrespective of their native expression levels in Msm to almost negligible levels in an ATc dose-dependent manner. Partial expression of YidC MS even after treatment with 10 ng ml −1 ATc for 24 h, however, could be due to either unstable dCas9–sgRNA hybridization to the target sequence or long half-life of YidC MS protein. To test these assumptions, we analysed YidC MS expression by increasing either the length of complementary sequence or time of incubation with ATc. It was found that increasing the length of hybridizing sequences to 25 bp results in 22% more suppression of YidC MS compared with its expression in Msm harbouring original construct with 20-bp complementary sequence ( Supplementary Fig. 4 ). In contrast, increasing the time of ATc incubation for additional 24 h does not cause any significant change in expression levels of YidC MS ( Supplementary Fig. 4 ). These results thus clearly demonstrate that a stable binding of dCas9 with the target DNA sequence is critical for silencing. Similar effects of CRISPRi were also noticed in slow-growing Mtb complex bacteria ( Fig. 5 ). In a systematic analysis, it was shown that yidC expression is gradually diminished in yidC(−) strain of BCG with increasing doses of ATc for 2 days ( Fig. 5a ). Remarkably, there was no effect of dCas9 overexpression on yidC in the control strain lacking yidC -specific sgRNA, which demonstrates a specific effect of dCas9 on sgRNA-mediated suppression of target genes. Importantly, prolonged incubation of the BCG cultures with ATc results in complete shutdown of YidC expression, and this effect is maintained for up to 1 week ( Fig. 5b ). Notably, a minor but consistent downregulation of GroEL1 was observed in yidC(−) strain ( Fig. 5b ). A comparative proteome analysis of the control and yidC(−) strains by isobaric tags for relative and absolute quantitation revealed that GroEL1 levels are indeed downregulated by fourfold in the knockdown strain compared with its expression in the control Mtb (P.T., unpublished observations). Similar to its effect in Msm and BCG, CRISPRi approach works with multiple genes of virulent Mtb that exhibit a wide range of expression levels ( Fig. 5c,d and Supplementary Table 3 ). In addition, we show that sgRNAs targeting the operon repress the downstream genes to a similar level ( Fig. 6 ). Overall, these results clearly demonstrate that CRISPRi approach is universally effective in targeted inactivation of genes irrespective of their native expression levels in both the fast- and the slow-growing mycobacteria. Although CRISPRi holds multiple implications, here we highlighted two major applications of this technique. We show that CRISPRi technique is useful in correctly identifying essential genes in mycobacteria ( Figs 4c–e and 5e ). Among several targets, the most interesting is yidC , which is predicted essential in all mycobacterial species. On the contrary, this study reveals differential requirements of YidC in the fast- and the slow-growing mycobacterial species ( Figs 4e and 5e ). Interestingly, a minor expression of YidC in the yidC MS (−) knockdown strain is sufficient to maintain bacterial growth in the synthetic culture media ( Fig. 4e ). These results also warrant further investigation of the role of the yidC MS in Msm by employing a conditional yidC MS deletion mutant. Two genes mmpL3 and ftsZ were used as reference controls that are essential for mycobacterial growth [35] , [36] . Next, we demonstrate that akin to its effect on a single target, CRISPRi is also competent in knocking-down the expression of multiple transcripts ( Fig. 7 ). Thus, the CRISPRi approach may be proven useful in understanding the function of redundant genes in mycobacteria. Even though CRISPRi is efficient in downregulating the expression of various genes in mycobacteria, an off-target effect of this approach cannot be completely ruled out. Hence, complementation with a wild-type copy will be critical in establishing function of a particular gene to associated phenotypes of the corresponding knockdown strain. Recent years have witnessed a sharp increase in the emergence of drug-resistant Mtb strains. To eradicate multidrug- and extensively drug-resistant TB cases, newer treatment options such as better vaccines and chemotherapeutic agents are immediately required. However, such goals cannot be achieved without characterizing proteins of unknown function. Our study provides a powerful tool to perform genetic manipulations for better understanding the functions of hitherto unknown proteins in Mtb, a pathogen which accounts for two deaths every 3 min (ref. 37 ). Culturing of bacteria In this study, we used E. coli strain DH5α, Msm mc 2 155, Mtb H37Rv and M. bovis BCG Pasteur, as described earlier [38] . Briefly, Mtb and BCG were cultured either in Middlebrook 7H9 broth supplemented with 1 × OADC, 0.02% tyloxapol and 0.5% glycerol or on Middlebrook 7H11 agar supplemented with 1 × OADC and 0.5% glycerol. Msm was cultured either in 7H9 broth containing 0.02% tyloxapol and 0.5% glycerol or on Middlebrook 7H11 agar supplemented with 0.5% glycerol, whereas E. coli was cultured in Luria-Bertani medium supplemented with appropriate antibiotics (50 μg ml −1 kanamycin or 150 μg ml −1 hygromycin), wherever needed. Bacteria were grown at 37 °C with (in broth) or without (on agar) shaking at 200 r.p.m. Cultures of mycobacterial cells harbouring pTetInt– dcas9 were maintained in the culture media containing 25 μg ml −1 kanamycin, whereas those co-transformed with pTetInt– dcas9 and pGrna were cultured in the presence of 25 μg ml −1 kanamycin and 50 μg ml −1 hygromycin. To repress a gene, Msm cultures were supplemented with desired ATc concentrations every 24 h, whereas Mtb or BCG cultures were treated with ATc at every 96 h. Cloning of complementary sequences in pGrna To achieve repression of a particular gene in mycobacteria, a 20-bp sequence immediately following the 5′-CCN-3′ was targeted, as exemplified in the Fig. 1c,d . The respective target-specific complementary oligonucleotides, CRISPR_UP and CRISPR_DN ( Supplementary Table 2 ) were synthesized, annealed and cloned at SphI and AclI sites, upstream to Cas9 handle sequence into pGrna. The recombinant pGrna plasmid containing a 20-bp complementary region was subsequently transformed into dCas9-overexpressing mycobacteria to create the respective knockdown strains. For simultaneous expression of multiple sgRNAs, the second sgRNA cassette was first PCR amplified using the respective pGrna clone as template and P myc1 tetO -specific forward primer tet 5′ and a reverse primer tet 3′, flanking the terminator ( Supplementary Table 2 and Supplementary Fig. 2 ). Subsequently, the amplicon was end-filled by using Klenow DNA polymerase and the blunt-ended PCR product was cloned downstream to the existing sgRNA cassette in the same orientation into the pGrna plasmid at the Klenow-filled HindIII site. Extraction of total RNA Total RNA was extracted from mycobacteria by disrupting cells in TRIzol reagent according to the manufacturer’s instructions (Invitrogen). Whole-genome expression analysis by microarray Microarray slides containing 13,768 oligonucleotides encompassing three sets of 3,924 genes of Mtb were commercially obtained (Microarrays Inc). For probe preparation, complementary DNA (cDNA) was prepared from 6 μg of total RNA from the test and the control strains of Mtb. For each hybridization, the cDNA probes labelled with alexa fluor 555 or alexa fluor 647 (Life Technologies) were used in pairs. Slides were scanned using a GenePix 4000A microarray scanner (Axon Instruments), and the resulting images were analysed using GenePix Pro 7.2.22 software (Axon Instruments), which yielded three data sets because of printing for each gene in triplicate. The mean fluorescence intensity of alexa fluor 555 and alexa fluor 647 for each of the spots was normalized against the overall intensity, and intensities above the baseline value of 500 were used to determine the change in expression levels. RT–PCR and mRNA quantification Bacterial total RNA was treated with RNase-free DNase I (Ambion) to remove traces of contaminating DNA, which was verified by 30 cycles of PCR followed by ethidium bromide-stained agarose gel analysis. Subsequently, cDNA was synthesized from total RNA and was subjected to either regular PCR for semiquantitative estimation by ethidium bromide-stained agarose gel electrophoresis or RT–PCR for quantitative estimation, typically as described earlier [38] . For semiquantitative estimation, PCR was carried out at 95 °C for 10 s, 55 °C for 15 s and 72 °C for 30 s, for a total of 23–30 cycles pertinent to different primer sets. For absolute quantification of mRNA, standard curves for the respective transcripts were prepared by performing PCR using SYBR green detection with known amounts of genomic DNA. Immunoblot analysis Bacterial whole-cell extracts were separated by SDS–polyacrylamide gel electrophoresis (SDS–PAGE), followed by electrotransfer to nitrocellulose membranes. Each blot was subsequently cut into two halves at around the position of 55-kDa marker protein and subjected to immunoblotting using specific test and control antibodies. Immunoblotting was performed by blocking the membrane with 1 × PBS containing 3% non-fat-dried milk (NFDM) for 1 h followed by overnight incubation at 4 °C with primary antibodies specific to mycobacterial proteins. Antibodies against YidC and EngA were raised by repeated immunization of rabbits with conjugated peptides SARTPRPGVRPKKRKR and GRREAVVQDIPGVT, respectively, (Genscript), whereas polyclonal anti-GroEL1 and anti-PknB IgG preparations were generously provided by Dr Vinay Nandicoori at the National Institute of Immunology, India. As primary antibodies in the immunoblotting experiments, we used a 5,000-fold dilution of anti-YidC and anti-EngA, a 10,000-fold dilution of anti-PknB and a 50,000-fold dilution of anti-GroEL1 in PBS containing 0.05% Tween-20 and 5% NFDM. Subsequently, membrane was washed 3 × with PBS containing 0.3% Tween-20 followed by 1 h of incubation with 10,000-fold dilution of horseradish peroxidase-conjugated IgG in PBS containing 0.05% Tween-20 and 3% NFDM (GE Healthcare). After 3–5 washes with PBS containing Tween-20, membrane was incubated with chemiluminescent substrates (Pierce) and signals were obtained by autoradiography. Accession codes: Gene expression data have been deposited in GEO database under the accession code GSE64135 . How to cite this article : Choudhary, E. et al . Gene silencing by CRISPR interference in mycobacteria. Nat. Commun. 6:6267 doi: 10.1038/ncomms7267 (2015).